Upper mantle viscosity and dynamic subsidence of curved continental margins Continental rifting does not always follow a straight line. Nevertheless, little attention has been given to the influence of rifting curvature in the evolution of extended margins. Here, using a three-dimensional model to simulate mantle dynamics, we demonstrate that the curvature of rifting along a margin also controls post-rift basin subsidence. Our results indicate that a concave-oceanward margin subsides faster than a convex margin does during the post-rift phase. This dynamic subsidence of curved margins is a result of lateral thermal conduction and mantle convection. Furthermore, the differential subsidence is strongly dependent on the viscosity structure. As a natural example, we analyse the post-rift stratigraphic evolution of the Santos Basin, southeastern Brazil. The differential dynamic subsidence of this margin is only possible if the viscosity of the upper mantle is >2–3 × 10 19 Pa s. The post-rift tectonic subsidence of divergent margins is mainly explained by the thermal contraction of a thinned lithosphere and its isostatic response to cooling due to vertical heat flow [1] , [2] in a one-dimensional model. Although lithospheric cooling is mainly guided by this vertical heat flow through the margin, two-dimensional (2D) numerical models [3] , [4] , [5] show that lateral thermal conduction has an important role in controlling the rate of subsidence. For the same amount of lithospheric stretching, a 2D model predicts faster subsidence than a one-dimensional model does [4] . A 2D model depends on the horizontal temperature gradient, which is a function of lateral variations in lithospheric thickness. Another important process that controls subsidence of the margin is mantle advection beneath the lithosphere [6] , [7] , which is also a function of mantle viscosity. Lateral variations in lithospheric thickness across the margin induce small-scale convection [8] , which increases heat transfer to the thinned lithosphere and adjacent areas [9] . One consequence of this process is a transient uplift of the flanks of the rift and a decrease in the subsidence rate of the adjacent stretched lithosphere [10] . In this case, the isostatic effect of the additional heat introduced into the stretched lithosphere due to the small-scale mantle convection acts against the subsidence caused by vertical and lateral heat conduction. Therefore, the cumulative subsidence depends on the competing effects of conductive and advective heat transport within the margin. Although previous 2D models of continental margin subsidence have shown the importance of incorporating a horizontal dimension and convective processes into the study of subsidence, little attention has been given to the influence of the assumed planar shape of the rifting, with a few exceptions [11] , [12] . Several portions of divergent marginal basins around the world have curved segments, and 2D models may not adequately describe their subsidence histories. Examples include the southeastern Brazilian margin and its conjugate, the western African margin. To study the thermal evolution of a stretched margin following rifting, we used the three-dimensional (3D) finite element code CitcomCU [13] , [14] to simulate convection in the upper 660 km of the Earth. Using different numerical simulations, we observe that the subsidence pattern of a curved margin is sensitive to the viscosity structure of the upper mantle. For a viscous upper mantle, the subsidence is mainly guided by the thermal conduction, which is more efficient in the concave segment of the margin than in the convex one. Therefore, a differential subsidence is expected along a curved margin. For a less-viscous upper mantle, the influence of advection in the thermal structure of the mantle becomes increasingly important and reduces the differential subsidence promoted by the thermal conduction. These concepts are applied to study the evolution of the southeastern Brazilian margin. Differential subsidence and upper mantle viscosity In our numerical simulations, we assumed a temperature- and pressure-dependent Newtonian rheology, with the viscosity η given by the Arrhenius law: where E and V are the (non-dimensional) activation energy and volume, respectively, z is depth, D is the thickness of the model, T is temperature, Δ T is the decrease in temperature from the base of the model to the surface, T 0 =0.21 is a non-dimensional constant and η 0 = η ( D, Δ T ) is the viscosity at the base of the model. The temperature profile is linear with depth to the base of the lithosphere, and the lithospheric stretching factor [2] β varies from 1 to 3 ( Fig. 1a ). This implies that the thickness of the thinned lithosphere is 1/ β of its original thickness. In plan view, the transition from the continent to the stretched margin is curved and contains a concave-oceanward segment and a convex segment ( Fig. 1b ). Additional information is found in the Methods section. 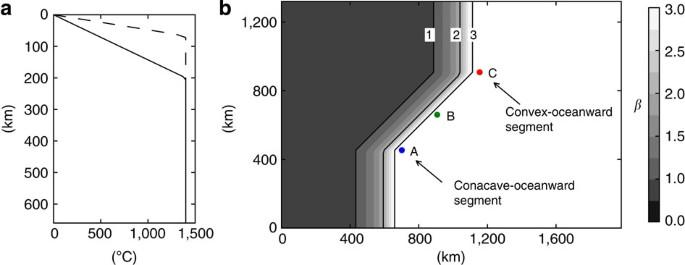Figure 1: Initial configuration of the numerical model. (a) Temperature profile for the unstretched continental lithosphere (solid line) and stretched lithosphere withβ=3 (dashed line). (b) Map of stretching factorβ, ranging from 1 to 3. The subsidence history of the margin is analysed at locations A, B and C withβ=3. We analysed the subsidence in three locations of the margin with β =3: location A is in the concave segment, location C is in the convex segment and location B is between locations A and C. Figure 1: Initial configuration of the numerical model. ( a ) Temperature profile for the unstretched continental lithosphere (solid line) and stretched lithosphere with β =3 (dashed line). ( b ) Map of stretching factor β , ranging from 1 to 3. The subsidence history of the margin is analysed at locations A, B and C with β =3. Full size image In the first simulation, for a mantle with η 0 =5 × 10 20 Pa s, E =30 and V =0 ( Fig. 2a , first column), the rate of subsidence decreases from the concave segment towards the convex segment (from A to C), and the difference in subsidence between locations C and A increases over time, reaching >250 m during the post-rift evolution of the margin when assuming a water-filled basin ( Fig. 2a , third column). This result implies that the subsidence is faster in the concave segment than in the convex segment during the post-rift phase, generating more space to accommodate the sediments in the concave segment. The load of the sediments filling this accommodation space triples the differential subsidence caused only by the water load. Despite the fact that the lithosphere has the same stretching factor at the three locations along the margin, the subsidence histories of these sites are distinct due to more efficient cooling of the stretched lithosphere through lateral conduction in the concave segment. In addition, the small-scale convection induced beneath the stretched lithosphere is more vigorous in the concave segment than for any other geometrical configuration, with advection beneath location A that is up to 70% faster than that under location C ( Fig. 2a , second column). Consequently, the heating of the margin by advection is more efficient at A than at C, reducing the difference in subsidence along the margin. However, because of the relatively high viscosity of the mantle in this case, the advection is slow ( Fig. 2a , second column), and the thermal evolution of the model is mainly guided by heat conduction. 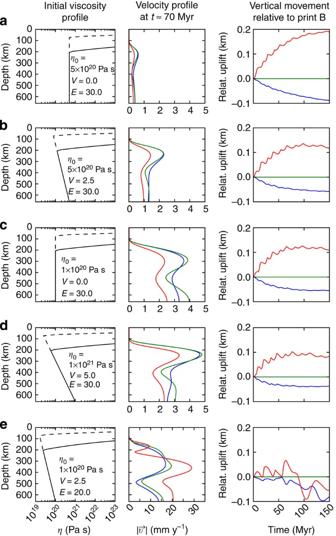Figure 2: Evolution of the margin for different viscosity structures. Letters a-e are different simulations. (first column) Initial viscosity profile for the continent (β=1, solid line) and stretched lithosphere (β=3, dashed line). (second column) Velocity profile for locations A (blue), B (green) and C (red) att70 Myr. (third column) Vertical movement of A (blue) and C (red) relative to B (green) over time assuming a water-filled basin. Figure 2: Evolution of the margin for different viscosity structures. Letters a-e are different simulations. (first column) Initial viscosity profile for the continent ( β =1, solid line) and stretched lithosphere ( β =3, dashed line). (second column) Velocity profile for locations A (blue), B (green) and C (red) at t 70 Myr. (third column) Vertical movement of A (blue) and C (red) relative to B (green) over time assuming a water-filled basin. Full size image Regardless of the location along the margin, the stretched lithosphere closer to the continent subsides faster than that farther from the continent. This more rapid subsidence persists over time during the evolution of the margin ( Supplementary Figs S1–S5 ). In the following simulations, we consider a less-viscous mantle ( Fig. 2b–d , first column), which causes small-scale convection to be more vigorous and advective heating to be more efficient. As in the first simulation, the advection under the concave segment is more vigorous than that under the convex segment ( Fig. 2b–d , second column). The influence of advective heat under the stretched margin with a lower-viscosity mantle reduces the differential subsidence along the margin promoted by lateral thermal conduction, resulting in 100–150 m of differential subsidence between locations A and C during the post-rift evolution of the margin ( Fig. 2b–d , third column) for a water-filled basin. The interaction of small-scale mantle convection with the lithosphere also produces oscillations in subsidence along the margin over periods of a few millions of years (Myr), with a peak-to-peak amplitude of a few metres to tens of metres. These oscillations are in addition to the increasing differential subsidence along the margin ( Fig. 2b–d , third column) and can be associated with the development of stratigraphic sequences [15] . The combined effect of small-scale mantle convection and thermal conduction in the 3D model predicts another important phenomenon: the modelled rate of relative subsidence along the margin does not reach its maximum in the initial stage of the process and decrease with time; instead, its maximum occurs after ~15–20 Myr ( Fig. 2b–d , third column). This result indicates that the post-rift differential subsidence along the margin may originate up to many millions of years after the end of the rifting phase. In addition, >70% of the differential subsidence occur during the first 50 Myr. Therefore, most of the differential subsidence occur ~15–50 Myr after the beginning of the simulation for models ( Fig. 2b–d ). For a less-viscous upper mantle with η <2–3 × 10 19 Pa s under the stretched margin ( Fig. 2e , first column), the subsidence of the margin does not depend on its position along the curved margin. Only oscillations related to the small-scale convection with amplitudes <100 m are observed ( Fig. 2e , third column). In this case, lateral heat conduction is overcome by vigorous advection ( Fig. 2e , second column; Supplementary Fig. S6 ). Therefore, the differential subsidence along the margin is strongly dependent on the viscosity of the upper mantle ( Fig. 3 ). 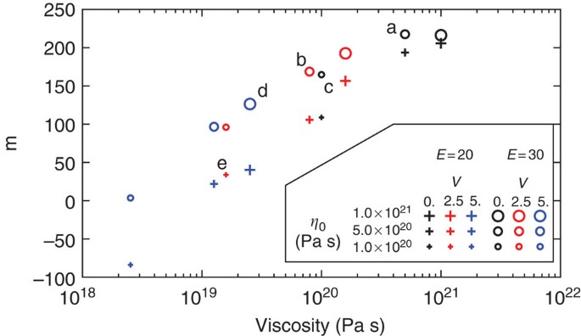Figure 3: Mean difference in subsidence between locations A and C. The mean difference in subsidence, taken for the time interval 50–100 Myr, is given as a function of the non-dimensional activation energyE, the non-dimensional activation volumeVand the viscosityη0. The viscosity indicated on the horizontal axis is at the base of the lithosphere. The letters a–e indicate the respective model inFig. 2. Figure 3: Mean difference in subsidence between locations A and C. The mean difference in subsidence, taken for the time interval 50–100 Myr, is given as a function of the non-dimensional activation energy E , the non-dimensional activation volume V and the viscosity η 0 . The viscosity indicated on the horizontal axis is at the base of the lithosphere. The letters a–e indicate the respective model in Fig. 2 . Full size image The influence of the lithospheric flexural rigidity To evaluate how the differential subsidence along a curved margin is affected when we account for the flexural rigidity of the lithosphere, we assume that a thin elastic plate represents the flexural behaviour of the lithosphere. In this case, the vertical deflection w of the lithosphere due to the vertical load q is given by the following equation: where E Y is Young’s modulus, T e is the effective elastic thickness, ν is Poisson’s ratio, and ρ m and ρ w are mantle and water density, respectively. Assuming a constant flexural rigidity D , we use a spectral method to determine the vertical deflection of the thin elastic plate [16] . We calculate the flexural response of the lithosphere for the models in Fig. 2a–e at t =70 Myr, with T e ranging from 0 to 39 km. Other constants of the model are E Y =10 11 Pa and ν =0.25. The vertical displacements of locations A and C relative to B are shown in Supplementary Fig. S7 . For the models in Fig. 2a–d where the differential subsidence was observed, the magnitude of the vertical deflection of the plate between the three locations does not change significantly for T e <15–20 km. Therefore, the flexural rigidity of the lithosphere also influences the magnitude of the differential subsidence, but this is only significant when the effective elastic thickness T e is large ( T e >15–20 km) because the viscous lithosphere naturally filters out short-wavelength stresses applied to its base [17] . In addition, the increase in flexural rigidity does not necessarily smooth differential subsidence, but it may eventually amplify differential subsidence due to the curved geometry of the margin [18] , [12] . To apply this 3D model to a curved margin, we analysed the stratigraphic evolution of the Santos Basin offshore of southeastern Brazil. This sedimentary basin originated in a stretched lithosphere with a geometrical configuration similar to that used in our numerical model ( Fig. 4 ). The southwestern portion of the basin lies on a concave-oceanward segment of the margin, whereas the northeastern portion is similar to a convex segment, with an estimated mean β 2.9 (ref. 19 ). The sedimentation in the Santos Basin has varied substantially along the margin over time (section in Fig. 4 ), and the depocentre migrated northeastward during the Cenomanian to Maastrichtian [20] (depositional sequences III–VII in Fig. 4 ). In particular, the Cenomanian-lower Turonian sedimentation was initiated nearly 23 Myr after the end of rifting and is limited by the Cenomanian and the intra-Turonian unconformities [21] . This sedimentation occurred mainly in the southwestern portion of the basin, with a present-day mean thickness of ~400–600 m ( Fig. 4 , III). The asymmetric sedimentation continued with lower magnitude in the upper Turonian-lower Santonian sedimentation ( Fig. 4 , IV), with the top limited by the Santonian unconformity [21] . This sedimentary pattern can be explained by the differential subsidence of the margin due to the combined effect of the 3D geometry and the dynamic evolution of the stretched margin, resulting in faster subsidence rates to the southwest during this period. A simple variation in the stretching factor β along the margin cannot explain the beginning of the differential subsidence many million years after the end of rifting. 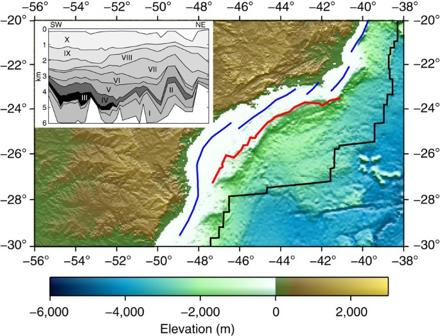Figure 4: Southeastern margin of Brazil and the offshore Santos Basin. The black curve shows the ocean–continent boundary, and the blue curves indicate the hinge zone that represents the western limit of significant continental extension34. The red curve indicates the location of the section shown in the upper-left corner of the figure with ~900 km in length. The section represents the lateral correlation of different depositional sequences extracted from 32 wells in the Santos Basin20. I: Lower Albian; II: Upper Albian; III: Cenomanian-lower Turonian; IV: Upper Turonian-lower Santonian; V: Upper Santonian-lower Campanian; VI: Upper Campanian; VII: Maastrichtian; XIII: Palaeocene-lower Oligocene; IX: Upper Oligocene-lower Miocene; and X: Upper Miocene-Present. The pre-Albian layers are not shown because of a lack of information and do not influence the conclusions of this work. Figure 4: Southeastern margin of Brazil and the offshore Santos Basin. The black curve shows the ocean–continent boundary, and the blue curves indicate the hinge zone that represents the western limit of significant continental extension [34] . The red curve indicates the location of the section shown in the upper-left corner of the figure with ~900 km in length. The section represents the lateral correlation of different depositional sequences extracted from 32 wells in the Santos Basin [20] . I: Lower Albian; II: Upper Albian; III: Cenomanian-lower Turonian; IV: Upper Turonian-lower Santonian; V: Upper Santonian-lower Campanian; VI: Upper Campanian; VII: Maastrichtian; XIII: Palaeocene-lower Oligocene; IX: Upper Oligocene-lower Miocene; and X: Upper Miocene-Present. The pre-Albian layers are not shown because of a lack of information and do not influence the conclusions of this work. Full size image To illustrate how the 3D geometry of the Brazilian margin influenced the subsidence of the Santos Basin, we constructed a numerical model with a simple margin geometry that resembles the southeastern Brazilian margin (see Methods). For this example, we used the viscosity structure of the model in Fig. 2c . From the numerical results, we calculated the total subsidence of the margin for the time interval equivalent to the Cenomanian to lower Santonian sedimentation in the Santos Basin after the end of rifting (Lower Aptian). Assuming a sediment-filled basin, the numerical model can predict the main pattern of sediment thickness along the Santos Basin deposited during this interval of time ( Fig. 5 ). Despite some discrepancies between the observed and calculated thicknesses, this example shows that the regional variations in the sedimentary thickness can be guided by the geometry of the margin combined with the mantle dynamics. 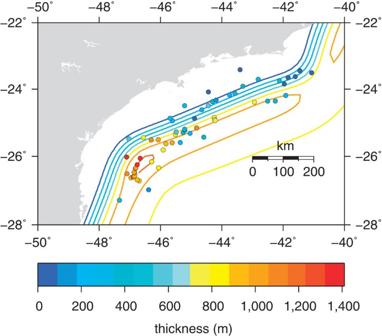Figure 5: Comparison between the observed and the predicted sedimentation. The dots indicate the observed thicknesses of the Cenomanian-lower Santonian sedimentation, and the curves show the sedimentation predicted by the numerical model. The sedimentary thicknesses were extracted from 61 wells in the Santos Basin20. The curves derived from the numerical model range from 0 to 1 200 m and are in intervals of 200 m, with the same colour scale of the well data. Figure 5: Comparison between the observed and the predicted sedimentation. The dots indicate the observed thicknesses of the Cenomanian-lower Santonian sedimentation, and the curves show the sedimentation predicted by the numerical model. The sedimentary thicknesses were extracted from 61 wells in the Santos Basin [20] . The curves derived from the numerical model range from 0 to 1 200 m and are in intervals of 200 m, with the same colour scale of the well data. Full size image The gliding of Aptian salt from the platform to the deep ocean created an additional accommodation space during the post-rift evolution of the Santos Basin and may hinder the quantification of differential subsidence produced by mantle dynamics. However, although the timing of salt gliding is not clearly known, previous studies suggest that the gliding occurred mainly during the Albian [22] , [23] , Santonian-Maastrichtian [24] and Palaeocene [25] . Therefore, the asymmetric Cenomanian-lower Santonian sedimentation could have been partially driven by the differential subsidence as a result of the margin curvature and the mantle dynamics. Later, the Santonian-Maastrichtian salt gliding may have contributed to the migration of the depocentre of the Santos Basin towards the northeast, with the additional contribution of varying sediment supply along the margin [26] ( Fig. 4 , IV–VII). In addition, previous estimates of T e for the southeastern Brazilian margin indicate that T e <20 km [27] , [28] . Therefore, based on our flexural analysis for different lithospheric flexural rigidities, the differential subsidence along the margin is not significantly modified for the low T e values observed in the southeastern Brazilian margin. The differential subsidence in the Santos Basin promoted by the curved geometry of the margin and mantle dynamics is only possible if the viscosity of the upper mantle under the margin is >2–3 × 10 19 Pa s. This lower limit for the viscosity is coherent with the viscosity obtained for other continental margins from the observation of sea-level variations due to glacial melting in the Upper Pleistocene and Holocene and the Earth’s consequent adjustment to the water load, indicating that the upper mantle viscosity beneath continental margins ranges between 10 20 and 10 21 Pa s (refs 29 , 30 ). Our study demonstrates how the integration of mantle dynamics and the use of a full 3D model in basin analysis may provide new insights into the physical properties of the mantle. This approach could be extended to other curved margins such as the Gulf of Guinea, northeastern Brazil and Angola margins. Model parameters and boundary conditions Using the finite element code CitcomCU, we constructed a 3D Cartesian box that is 660 km deep, 1,320 km wide and 1,980 km long, with 65 × 65 × 97=409,825 nodes. The initial thermal structure follows the scheme shown in Fig. 1 . The temperatures at the surface and base of the model were held constant at T =0 and 1,400 °C, respectively. To improve the numerical stability, we imposed an upper limit for the viscosity of η ≤2.0 × 10 25 Pa s, which is similar to the maximum cut-off value for the viscosity used in previous works [31] , [32] . As boundary conditions, we assumed free slip at the top and at the bottom and reflecting sidewalls. Other parameters used in the numerical model are shown in Table 1 . Table 1 Parameters of the numerical model. Full size table Numerical model for the Brazilian margin To adequately simulate the subsidence of the Brazilian margin, we constructed a model very similar to the model shown in Fig. 1 with the only difference that the transition from β =1 to β =3 is narrower, with nearly half of the width of the transition shown in Fig. 1 . In addition, the model shown in Fig. 5 was rotated 24° clockwise. The viscosity structure of the model is the same as that of the model shown in Fig. 2c : η 0 =1 × 10 20 Pa s, E =30 and V =0. In this simulation, the total subsidence of the margin was calculated relative to the interior of the continent, specifically the node at the corner of the model in ( x,y )=(0,0) (see Fig. 1 ). How to cite this article: Sacek, V. and Ussami, N. Upper mantle viscosity and dynamic subsidence of curved continental margins. Nat. Commun. 4:2036 doi: 10.1038/ncomms3036 (2013).